A sequence-specific DNA glycosylase mediates restriction-modification inPyrococcus abyssi Restriction-modification systems consist of genes that encode a restriction enzyme and a cognate methyltransferase. Thus far, it was believed that restriction enzymes are sequence-specific endonucleases that introduce double-strand breaks at specific sites by catalysing the cleavages of phosphodiester bonds. Here we report that based on the crystal structure and enzymatic activity, one of the restriction enzymes, R.PabI, is not an endonuclease but a sequence-specific adenine DNA glycosylase. The structure of the R.PabI–DNA complex shows that R.PabI unwinds DNA at a 5′-GTAC-3′ site and flips the guanine and adenine bases out of the DNA helix to recognize the sequence. R.PabI catalyses the hydrolysis of the N -glycosidic bond between the adenine base and the sugar in the DNA and produces two opposing apurinic/apyrimidinic (AP) sites. The opposing AP sites are cleaved by heat-promoted β elimination and/or by endogenous AP endonucleases of host cells to introduce a double-strand break. Restriction enzymes recognize specific DNA sequences and introduce strand breaks, unless the sequences are methylated by the cognate methyltransferases [1] . In prokaryotic cells, restriction-modification systems limit transfers of exogenous DNA and protect against infection by phages. In addition, there is some evidence that certain restriction-modification gene complexes act as selfish mobile elements in the manner of viral genomes and transposons [2] , [3] —that is, they limit the movements of genes, but are themselves mobile. It has generally been thought that restriction enzymes are sequence-specific endonucleases that expose the 3′-OH end and 5′-phosphate end. In the field of biotechnology, type II restriction enzymes, which introduce a strand break at or near their recognition sequence, are frequently used to cut DNA duplexes at specific sites in order to manipulate and analyse DNA. Most of the type II restriction enzymes whose nuclease activities have been experimentally confirmed use Mg 2+ ions for these nuclease activities and have a PD-(D/E)XK motif in their active sites [4] , [5] , [6] . Other type II restriction enzymes belong to the phospholipase D (PLD) superfamily, the HNH superfamily and the GIY-YIG superfamily [6] , [7] , [8] , [9] , [10] . In addition to these restriction enzyme superfamilies, we found a half-pipe superfamily for which R.PabI from the hyperthermophilic archaea Pyrococcus abyssi is representative [11] , [12] . There is no protein with a structure similar to the overall fold of R.PabI [12] . R.PabI is a type II restriction enzyme that has a novel DNA-binding fold called a ‘half-pipe,’ which consists of a highly curved anti-parallel β-sheet ( Fig. 1a ). R.PabI recognizes a 5′-GTAC-3′ sequence and cleaves DNA duplexes at high temperature without the addition of a divalent cation, although restriction enzymes generally require Mg 2+ ions for their enzymatic activities (the sole exception is restriction enzymes for the PLD superfamily [7] ). Among the thousands of confirmed and hypothetical restriction enzymes identified, only a few proteins are predicted to have the half-pipe fold [6] . Recent genomic analyses have revealed that R.PabI homologues are found in some mesophilic bacteria, such as Helicobacter and Campylobacter , in a thermophilic bacterium ( Caloramator australicus ), and in some hyperthermophilic archaea ( Acidilobus saccharovorans and Staphylothermus hellenicus ) ( Supplementary Fig. 1 ). Among these homologues, it has been experimentally confirmed that the R.PabI homologue in H. pylori R.HpyAXII also cleaves the 5′-GTAC-3′ sequence and limits exogenous DNA uptake [13] . The structural and mutational analyses of R.PabI in our previous work showed that R.PabI forms a homodimer and recognizes DNA duplexes using its electropositive half-pipe region [12] , but the structural basis of the sequence-recognition and DNA-cleavage mechanisms were still unclear because the structure of the R.PabI–DNA complex had not been determined. 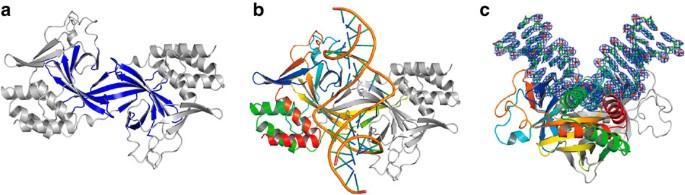Figure 1: Overall structure of the R.PabI–DNA complex. (a) Ribbon diagram of R.PabI. The characteristic half-pipe region is coloured blue. (b) Ribbon diagram of the R.PabI–DNA complex. The ribbon of one R.PabI protomer is coloured blue (in the N terminus) to red (in the C terminus). The other R.PabI protomer is coloured grey. The bound DNA is coloured orange. (c) Side view ofb. The composite omit map of the bound DNA is contoured at 2 σ (blue mesh). The structure of DNA is shown using a stick model. Figure 1: Overall structure of the R.PabI–DNA complex. ( a ) Ribbon diagram of R.PabI. The characteristic half-pipe region is coloured blue. ( b ) Ribbon diagram of the R.PabI–DNA complex. The ribbon of one R.PabI protomer is coloured blue (in the N terminus) to red (in the C terminus). The other R.PabI protomer is coloured grey. The bound DNA is coloured orange. ( c ) Side view of b . The composite omit map of the bound DNA is contoured at 2 σ (blue mesh). The structure of DNA is shown using a stick model. Full size image Here we report the crystal structure of the restriction enzyme R.PabI in complex with a DNA duplex containing the R.PabI recognition sequence. Our structural and biochemical analyses revealed that R.PabI is not an endonuclease that cleaves a sugar–phosphate backbone, but a sequence-specific DNA glycosylase that excises an adenine base. DNA glycosylases are a family of enzymes that are involved in base excision repair and catalyse the removal of damaged bases [14] , [15] , [16] . However, a DNA glycosylase that recognizes not a damaged base but a base in a specific DNA sequence and that acts as a dimer has never been reported. In addition, there has been no report of a restriction enzyme that exhibits DNA glycosylase activity. Our results demonstrate the mechanism by which R.PabI uses DNA glycosylase activity for sequence-specific DNA cleavage. Overall structure of the R.PabI–DNA complex To determine the crystal structure of the R.PabI–DNA complex, we used the R.PabI K154A mutant, which shows reduced DNA-cleavage activity ( Supplementary Fig. 2 ). We determined the crystal structure of the R.PabI K154A–DNA complex at 3.0 Å resolution by X-ray crystallography ( Fig. 1 and Supplementary Fig. 3 ). The asymmetric unit of the crystal contains one R.PabI–DNA complex that is composed of two R.PabI protomers (protomers A and B) and a DNA duplex. As predicted in our previous work [12] , the R.PabI dimer binds to the 5′-GTAC-3′ sequence using its half-pipe region. R.PabI bends the DNA duplex by ~90°, and the highly expanded minor groove side of the bended DNA faces the half-pipe region. The structure of R.PabI is slightly modified from the substrate-free form to accommodate the bended DNA duplex ( Supplementary Fig. 4 ). When the structure of R.PabI in complex with the DNA duplex is compared with that of the substrate-free form [12] , the structure of each protomer is slightly twisted in a counterclockwise direction and the β8–β9 loop sticks out toward the bound DNA. Interestingly, in the R.PabI–DNA complex, the DNA duplex of the 5′-GTAC-3′ site is unwound by the binding of R.PabI ( Fig. 1b ). The β8–β9 loop invades the DNA duplex from the highly expanded minor groove side to disrupt inter-base-pair hydrogen bonds of the recognition sequence and extrudes two purine bases (Gua9 and Ade11) from the DNA helix ( Fig. 2a ). The flipped guanine base is inserted into a pocket surrounded by Ser29, Lys30, Arg32, Glu63, Gln65, Lys152 and Tyr165, and is recognized by six hydrogen bonds with Ser29, Lys30, Glu63 and Lys152 ( Supplementary Fig. 5a,b ). The flipped adenine base is accommodated in a pocket surrounded by Ile66, Tyr68, Met163, Val164, Phe204 and His211, and is recognized by three hydrogen bonds with the main chain atoms of Ile66 and Val164 ( Supplementary Fig. 5c,d ). The inserted β8–β9 loop wraps the remaining Thy10 and Cyt12 and fills the space between the DNA strands to stabilize the unwound DNA structure. The pyrimidine rings of Thy10 and Cyt12 stack with each other due to the flipping out of the Ade11 nucleoside and are sandwiched by Arg156 and Met163. These bases are recognized by six hydrogen bonds with Gln155, Arg156, Ala157 and Gln161 ( Supplementary Fig. 5e,f ). In addition to the sequence-specific interactions, the characteristic structure of each DNA strand is stabilized by eighteen hydrogen bonds between R.PabI and the DNA backbone ( Supplementary Figs 5,6 ). The intermolecular hydrogen bonds between R.PabI and the DNA duplex are summarized in Fig. 2b and Supplementary Table 1 . Sharp bending of the DNA duplex and base flipping are also observed in the structures of DNA glycosylases and AP site-specific endonucleases [17] , [18] , [19] , [20] , [21] , [22] . In addition, some type II restriction endonucleases also flip a base out of the DNA helix to optimize protein–DNA interactions [23] , [24] , [25] . However, the unwinding of the DNA duplex across four base-pairs and the flipping of two purine bases observed in the R.PabI–DNA complex are novel DNA capture mechanisms by DNA-binding proteins ( Supplementary Discussion and Supplementary Fig. 7 ). 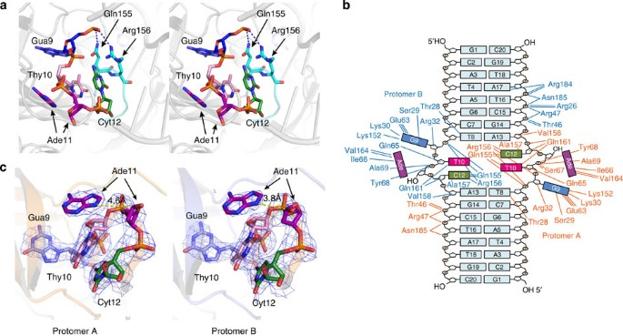Figure 2: R.PabI–DNA interaction. (a) Stereo view of the unwound DNA. Guanine, thymine, adenine and cytosine bases of the R.PabI recognition sequence are shown using blue, pink, purple and green stick models, respectively. R.PabI residues of the β8–β9 loop are shown using a cyan stick model. Hydrogen bonds are indicated by blue dotted-lines. (b) Intermolecular hydrogen bonds between R.PabI and the DNA duplex. The hydrogen bonds are indicated with lines. Residues from R.PabI protomers A and B are indicated by orange and blue, respectively. (c) The composite omit map (2 σ) around the R.PabI recognition sequence is shown by blue mesh. The structure of the R.PabI–DNA complex is shown using a stick model. Figure 2: R.PabI–DNA interaction. ( a ) Stereo view of the unwound DNA. Guanine, thymine, adenine and cytosine bases of the R.PabI recognition sequence are shown using blue, pink, purple and green stick models, respectively. R.PabI residues of the β8–β9 loop are shown using a cyan stick model. Hydrogen bonds are indicated by blue dotted-lines. ( b ) Intermolecular hydrogen bonds between R.PabI and the DNA duplex. The hydrogen bonds are indicated with lines. Residues from R.PabI protomers A and B are indicated by orange and blue, respectively. ( c ) The composite omit map (2 σ) around the R.PabI recognition sequence is shown by blue mesh. The structure of the R.PabI–DNA complex is shown using a stick model. Full size image The most striking feature of the R.PabI–DNA complex is that the electron density map of the N -glycosidic bond between the adenine base and deoxyribose of Ade11 is not observed ( Fig. 2c ). During the structure determination of the R.PabI–DNA complex, we observed an electron density corresponding to adenine apart from the DNA sugar–phosphate backbone. This suggests that R.PabI catalysed the cleavage of the N- glycosidic bond of Ade11 in the same way as DNA glycosylases during the co-crystallization experiment, and the structure determined in this study represents the R.PabI product DNA complex. It was also surprising that the DNA duplex containing two opposing AP sites was not cleaved ( Fig. 2c ), although AP sites are generally unstable and readily generate stand breaks. This suggests that, in the crystalline state, the unstable AP sites are stabilized by intermolecular contacts between R.PabI and the DNA duplex. DNA glycosylase assay The structural analysis of the R.PabI–DNA complex indicates that R.PabI catalyses the cleavage of the N -glycosidic bond in a manner similar to DNA glycosylases, although R.PabI shares no structural similarity to any DNA glycosylase. To confirm the adenine DNA glycosylase activity of R.PabI, we analysed the enzymatic activity of R.PabI in vitro . When a 5′-GTAC-3′-containing DNA duplex ( Supplementary Fig. 8a ) was treated with a different amount of R.PabI at 40 °C for 1 h, cleavages of oligonucleotides were detected by the addition of NaOH to the R.PabI products ( Fig. 3a ). These data indicate that R.PabI does not exhibit the DNA-cleavage activity at 40 °C, but does have the ability to produce AP sites on the substrate DNA at this temperature, because the AP sites generated by DNA glycosylases were unstable and were easily cleaved by NaOH treatment at the 5′ and 3′ side of the AP sites. Although 0.2 μM of the substrate DNA was almost completely cleaved by 0.4 μM of R.PabI dimer within 1 min ( Supplementary Fig. 8b ), an equal amount of substrate DNA was not completely cleaved by long-term incubation with 0.1 or 0.2 μΜ of R.PabI dimers ( Fig. 3a ). These data suggest that R.PabI forms a tight complex with the product DNA much like DNA glycosylases. The enzymatic rate constant and its standard error for removal of an adenine base, k obs , was estimated to be 4.5±0.1 min −1 . To confirm the sequence specificity of R.PabI, we performed a DNA glycosylase assay using closely related sequences as substrates ( Fig. 3b ). The results showed that R.PabI utilized the 5′-GTAC-3′ containing DNA duplex and the 5′-GTAC-3′ sequence of the mismatched DNA duplex as substrates. In addition, R.PabI also showed low DNA glycosylase activities for the 5′-CTAC-3′ sequence of the 5′-CTAC/CATG-5′ mismatch and the single-stranded DNA containing the 5′-GTAC-3′ sequence. 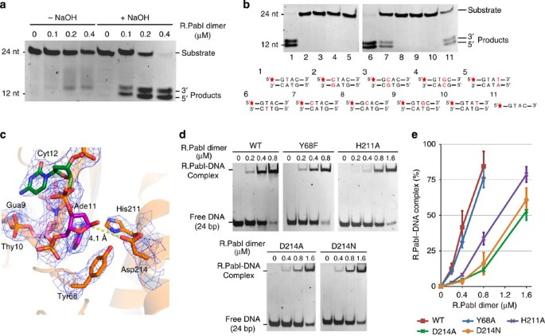Figure 3: Adenine DNA glycosylase activity and sequence-specific DNA binding of R.PabI. (a) DNA glycosylase assay as a function of increasing amounts of R.PabI at 40 °C. Half of the reaction was treated with NaOH to generate strand breaks at abasic sites. (b) Sequence specificity of R.PabI. DNA glycosylase assays were performed using closely related substrates at 40 °C. Lane 1: control; lanes 2–5: DNA duplexes with one-base substitution; 6–10: mismatched DNA duplexes with 5′-GTAC-3′ on one strand; 11: single-stranded DNA with the 5′-GTAC-3′ sequence. The position of the fluorescein label is indicated by a red star. (c) Active site structure of R.PabI. Conserved residues around Ade11 are shown using a stick model. The composite omit map (1.5 σ) is shown by blue mesh. (d) EMSA analyses of the wild-type R.PabI and its mutants. Fluorescein-labelled DNA duplex (0.2 μM) and R.PabI (0–1.6 μM) dimer were mixed and loaded on a 12% polyacrylamide gel. (e) Quantification ofd. Error bars represent the s.d. (n=3). Figure 3: Adenine DNA glycosylase activity and sequence-specific DNA binding of R.PabI. ( a ) DNA glycosylase assay as a function of increasing amounts of R.PabI at 40 °C. Half of the reaction was treated with NaOH to generate strand breaks at abasic sites. ( b ) Sequence specificity of R.PabI. DNA glycosylase assays were performed using closely related substrates at 40 °C. Lane 1: control; lanes 2–5: DNA duplexes with one-base substitution; 6–10: mismatched DNA duplexes with 5′-GTAC-3′ on one strand; 11: single-stranded DNA with the 5′-GTAC-3′ sequence. The position of the fluorescein label is indicated by a red star. ( c ) Active site structure of R.PabI. Conserved residues around Ade11 are shown using a stick model. The composite omit map (1.5 σ) is shown by blue mesh. ( d ) EMSA analyses of the wild-type R.PabI and its mutants. Fluorescein-labelled DNA duplex (0.2 μM) and R.PabI (0–1.6 μM) dimer were mixed and loaded on a 12% polyacrylamide gel. ( e ) Quantification of d . Error bars represent the s.d. ( n =3). Full size image The R.PabI products were also analysed by high-performance liquid chromatography (HPLC) and matrix-assisted laser desorption-ionization time-of-flight mass (MALDI-TOF MS) spectrometry. The results of the HPLC analyses showed that R.PabI was able to release adenine from the substrate DNA ( Supplementary Fig. 9 ). In addition, when the product DNA was analysed by MALDI-TOF MS spectrometry, a compound whose molecular weight was consistent with the hydrolyzed substrate DNA between adenine base and sugar in DNA was detected ( Supplementary Fig. 10 ). These results are consistent with the observation of the R.PabI–DNA complex structure. We conclude that R.PabI is a sequence-specific adenine DNA glycosylase. Mutation analysis of R.PabI In general, DNA glycosylases are classified into mono- or bifunctional enzymes based on their catalytic mechanisms. Most monofunctional DNA glycosylases have conserved carboxylate residues in the active site and catalyse hydrolysis of the N -glycosidic bond by a two-step dissociative pathway with an oxocarbenium cation intermediate [26] , [27] , [28] . On the other hand, bifunctional DNA glycosylases catalyse the removal of damaged bases and the cleavages of the sugar–phosphate backbone at AP sites via a Schiff base enzyme–DNA covalent intermediate using a conserved lysine or N-terminal proline residue in the active sites [29] , [30] , [31] . Because R.PabI does not show DNA-cleavage activity at 40 °C and contains Asp214 near the cleaved Ade11 ( Fig. 3c ), R.PabI would catalyse the hydrolysis of the N -glycosidic bond of Ade11 in a manner similar to monofunctional DNA glycosylases. In addition to Asp214, R.PabI has highly conserved Tyr68 and His211 residues near Asp214 ( Supplementary Fig. 1b ). Monofunctional DNA glycosylases have hydrophilic residues near the conserved carboxylate residues, such as arginine (alkyladenine DNA glycosylase [32] ) and asparagine (adenine DNA glycosylase [33] ), to stabilize the catalytic water molecule. Tyr68 and His211 of R.PabI might play the same role as these residues. Although the arrangement of Tyr68, His211, Asp214 and the hydrolyzed Ade11 shows no structural similarity to the active site structures of the known DNA glycosylases, these residues would be important for the DNA glycosylase activity of R.PabI. To determine the importance of these residues for the catalytic mechanism of R.PabI, we produced mutants of these residues and analysed their DNA glycosylase activities and DNA-binding affinities. The kinetic assay of the mutants showed that mutations of Y68F, D214A and D214N resulted in dramatic (~100 fold) decreases in the adenine release rates ( Table 1 and Supplementary Fig. 8b ). The reduced activities of the Y68F and D214N mutants suggest that the hydroxyl group of Tyr68 and the negative charge of Asp214 are important for the catalysis. In addition, the enzymatic activity of the H211A mutant was also reduced (~10 fold) ( Table 1 and Supplementary Fig. 8b ). In the R.PabI–DNA complex, the ND1 nitrogen of His211 forms a hydrogen bond with the hydroxyl group of Tyr68. His211 might be important for the localization of the hydroxyl group of Tyr68 in the active site. The DNA-binding affinity of each mutant is shown in Fig. 4d,e . Among the mutants, only the Y68F mutant showed the same DNA-binding affinity as the wild-type R.PabI. In contrast, the DNA-binding affinities of H211A, D214A and D214N were reduced. Because His211 constitutes a part of the adenine-binding pocket, the mutation to alanine would disrupt the adenine recognition mechanism of R.PabI. In the R.PabI–DNA complex, Asp214 does not undergo any interaction with the bound product DNA. Asp214, therefore, most likely is involved in binding to the substrate DNA. Table 1 Adenine DNA glycosylase activities of the wild-type R.PabI and its mutants. 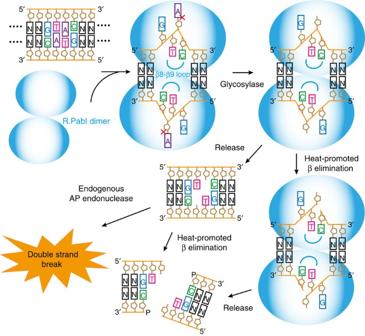Figure 4: DNA cleavage mechanism by R.PabI. Proposed DNA-cleavage mechanism by R.PabI. The opposing AP sites generated by R.PabI are cleaved by heat-promoted β elimination and/or endogenous AP endonucleases of host cells. Full size table Figure 4: DNA cleavage mechanism by R.PabI. Proposed DNA-cleavage mechanism by R.PabI. The opposing AP sites generated by R.PabI are cleaved by heat-promoted β elimination and/or endogenous AP endonucleases of host cells. Full size image In this study, we have revealed that R.PabI is a monofunctional adenine DNA glycosylase based on structural and biochemical analyses. Because the residues involved in the base recognition mechanisms and the DNA glycosylase activity are highly conserved among the R.PabI homologues ( Supplementary Fig. 1b,c ), the homologues appear to act as 5′-GTAC-3′-sequence-specific adenine DNA glycosylases. However, R.PabI and its homologues can cleave the DNA duplex at a specific site in a manner similar to restriction endonucleases [11] , [12] , [13] . In addition, the evidence that the expression of R.PabI is lethal for E. coli indicates that R.PabI acts as a restriction enzyme in living cells [12] . It is also known that the R.PabI homologue from H. pylori , R.HpyAXII, limits exogenous DNA uptake [13] . The opposing AP sites generated by R.PabI may be cleaved by two different mechanisms to introduce a double-strand break ( Fig. 4 ). First, the DNA strand treated by R.PabI is cleaved by heat-promoted β elimination ( Supplementary Figs 10b and 11a ). Because R.PabI is an enzyme from hyperthermophilic archaea, R.PabI shows DNA-cleavage activity at temperatures ranging from 60 °C to 90 °C (ref. 11 ). Under these conditions, the DNA duplex treated by R.PabI will be cleaved by heat-promoted β elimination at the AP sites. R.PabI homologues from thermophiles and hyperthermophiles would also cleave the DNA duplex by this mechanism. Second, the AP sites generated by R.PabI are cleaved by the AP endonucleases of host cells. Although R.PabI did not cleave the substrate DNA at 37 °C, the mixture of R.PabI and E. coli lysate cleaved the substrate DNA at the specific site ( Supplementary Fig. 11b ). These data suggest that R.PabI cooperates with endogenous nucleases to introduce a double-strand break at the specific site. Because H. pylori , which possess the R.PabI homologous enzyme R.HpyAXII, grow at a temperature around 37 °C, this cooperating mechanism would be important for R.HpyAXII to cleave exogenous DNA in H. pylori . Because the DNA fragments cleaved by R.PabI lose adenine bases at the cleavage site ( Fig. 4 ), it would be hard to re-ligate the R.PabI products, unlike in the case of DNA fragments produced by typical restriction endonucleases. This feature may make the restriction-modification system using DNA glycosylase activity more powerful in attacking DNA than the typical restriction-modification system. This is consistent with the fact that R.PabI homologues are frequently observed in Helicobacter , which is naturally competent for genetic transformation ( Supplementary Fig. 1 ) [34] . To date, six structural superfamilies of DNA glycosylases have been identified [16] . As R.PabI shares no structural similarity to known DNA glycosylases, the half-pipe superfamily represented by R.PabI is a new superfamily of DNA glycosylases. As shown in Fig. 3b , R.PabI could function as a strand-specific nicking enzyme on the mismatched duplex. Our results also raise the possibility that a novel DNA glycosylase that possesses a half-pipe fold might be discovered in a future study. Protein expression and purification The R.PabI K154A mutant, which contains 8–226 residues (R.PabI(K154A)), was used for the co-crystallization of R.PabI and DNA. The gene fragment of this construct was cloned into the pET26b vector (Novagen) and the constructed plasmid was transformed into E. coli Rosetta(DE3)pLysS (Novagen) for protein expression. The recombinant E. coli cells that overexpressed the R.PabI(K154A) were resuspended in 50 mM MES (pH 6.0) and 1 mM MgCl 2 and lysed by sonication. After centrifugation at 40,000 g for 30 min, the supernatant was treated with Cryonase Cold-active Nuclease (TAKARA) to remove contaminant DNA from E. coli , and heated at 80 °C for 30 min to denature heat-labile E. coli proteins. After centrifugation at 40,000 g for 30 min, the supernatant was applied onto a Toyopearl AF-Heparin-650M (TOSOH) column equilibrated with 50 mM MES (pH 6.0) and 300 mM NaCl. The R.PabI(K154A) was eluted with 50 mM MES (pH 6.0) and 1 M NaCl. The R.PabI(K154A) was further purified using a Resource S (GE Healthcare) column pre-equilibrated with 10 mM MES (pH 6.0) and was eluted with a linear gradient of 0–1 M NaCl. The gene fragments of the wild-type R.PabI and its mutants, which were used for the biochemical assays, were cloned into the pET28a vector (Novagen). The wild-type R.PabI was co-expressed with CviQI methyltransferase from chlorella virus NY-2A (M.CviQI), which methylates 5′-GTAC-3′, in E. coli BL21(DE3). The H211A mutant was co-expressed with M.CviQI in E. coli Rosetta(DE3)pLysS. The Y68F, K154A, D214A and D214N mutants were overexpressed in E. coli Rosetta(DE3)pLysS. The E. coli cells that overexpressed the wild-type R.PabI and its mutants were resuspended in 50 mM Tris–HCl (pH 8.0) and 10 mM imidazole and lysed by sonication. After centrifugation at 40,000 g for 30 min, the supernatant was applied onto an Ni-NTA Superflow (QIAGEN) column equilibrated with 50 mM Tris–HCl (pH 8.0) and 10 mM imidazole. The wild-type R.PabI and its mutants were eluted with 50 mM Tris–HCl (pH 8.0) and 200 mM imidazole. The wild-type R.PabI and its mutants were further purified using a Resource S column pre-equilibrated with 10 mM MES (pH 6.0) and eluted with a linear gradient of 0–1 M NaCl. Each purified protein was dialyzed against 10 mM MES (pH 6.0), 300 mM NaCl and 10 mM MgCl 2 and stored at −80 °C until use. Crystallization and structure determination For the co-crystallization of the R.PabI(K154A)–DNA complex, the purified R.PabI and a solution of 20-bp of a blunt-ended DNA duplex containing the R.PabI recognition sequence (5′-GCATAGCT GTAC AGCTATGC-3′; the R.PabI recognition sequence is underlined) were mixed at a molar ratio of 1:1 and concentrated to 185 μM. Crystallization experiments of the R.PabI–DNA complex were performed using the sitting-drop vapor-diffusion method at 20 °C. The crystals of the R.PabI–DNA complex were obtained in a reservoir solution containing 2.1 M sodium malonate (pH 7.0). X-ray diffraction data were collected on the AR-NE3A beamline at the Photon Factory (Tsukuba, Japan) under cryogenic conditions (95 K). The wavelength was set to 1.0 Å. The crystal of the R.PabI–DNA complex diffracted X-rays to 3.0 Å. X-ray diffraction data were indexed and integrated using the programme XDS [35] and scaled with SCALA in the CCP4 suite [36] . The crystal of the R.PabI–DNA complex belongs to the space group I 222 with unit cell parameters of a =104.51, b =151.40 and c =187.70 Å. The initial model of the R.PabI–DNA complex was determined by the molecular replacement method using the programme MOLREP [37] with the coordinates of the DNA-free R.PabI structure (PDB code: 2DVY) [12] . The initial model was refined and rebuilt using the programmes Phenix.refine [38] and Coot [39] . The final model of the R.PabI–DNA complex was refined to 3.0 Å resolution with R and R free values of 16.9% and 19.4%, respectively. The geometry of the final model was evaluated using the programme MolProbity [40] . In the Ramachandran plot, 97.0% of the residues were included in the favored region and the rest of the residues were in the allowed region. The data collection and refinement statistics are summarized in Table 2 . The structure of the R.PabI–DNA complex was depicted using the programme Pymol [41] . Intermolecular interactions between R.PabI and the DNA duplex were analysed using the programme PISA [42] . The composite omit map was generated using the CCP4 suite [36] . Table 2 Summary of data collection and refinement statistics of the R.PabI–DNA complex. Full size table DNA glycosylase assay Excision of adenine was detected by incubating R.PabI with the 5′-fluorescein-labelled 24-mer DNA duplex (5′-fluorescein-GGATGCATGA GTAC GAGGACCATC-3′) and following the appearance of the abasic DNA product after alkaline cleavage. For enzymatic reactions, 0.2 μM of the labelled DNA and 0.1–0.4 μM of R.PabI dimer were mixed in 10 μl of a reaction buffer containing 0.1 M sodium phosphate buffer (pH 6.5) and incubated at 40 °C for 1 h. Half of the total volume of each product was treated with 0.1 M NaOH, incubated at 70 °C for 10 min and neutralized by the addition of an equal amount of HCl. The solutions were separated through a denaturing 18% polyacrylamide gel in 0.5 × TBE and 7 M urea, and fluorescence was measured by an LAS4000 Mini system (Fujifilm, Tokyo, Japan). To analyse the sequence specificity of R.PabI, the closely related DNA duplexes (the 5′-GTAC/CATG-5′ site of the labelled DNA duplex described above was replaced with the 5′-CTAC/GATG-5′, 5′-GCAC/CGTG-5′, 5′-GTGC/CACG-5′, 5′-GTAT/CATA-5′, 5′-GTAC/CTTG-5′, 5′-CTAC/CATG-5′, 5′-GCAC/CATG-5′, 5′-GTGC/CATG-5′ and 5′-GTAT/CATG-5′ duplexes) and the 5′-fluorescein-labelled single-stranded DNA with the sequence described above were also utilized as substrates. For the enzymatic reactions, 0.2 μM of the labelled DNA and 0.4 μM of R.PabI dimer were mixed in 10 μl of a reaction buffer containing 0.1 M sodium phosphate buffer (pH 6.5) and incubated at 40 °C for 1 h. The products were treated with NaOH and separated through a denaturing 18% polyacrylamide gel as described above. The enzymatic rate constant k obs for the removal of adenine was determined by mixing 0.2 μM of the labelled DNA and 0.4 μM of R.PabI dimer in 10 μl of 0.1 M sodium phosphate buffer (pH 6.5) and incubating at 40 °C. To determine the level of base removal, the reactions were stopped at selected time points by adding NaOH to 0.1 M, and the products were separated through a denaturing 18% polyacrylamide gel as described above. The R.PabI products were quantified based on the fluorescence of the fluorescein. The enzymatic rate constant k was obtained from a single-exponential fit to the data from four independent measurements: f p =1–e – kt , in which f p is the fraction of product and t is the time of the reaction. HPLC assay To detect the production of free adenine by R.PabI treatment, the DNA duplex that was used for the co-crystallization was treated with R.PabI. For the R.PabI reaction, 50 μM of the substrate DNA and 25 μM of the R.PabI dimer were mixed in 200 μl of 10 mM MES (pH 6.0), 300 mM NaCl and 10 mM MgCl 2 and incubated at 40 °C for 30 min. To dissociate the R.PabI–DNA complex, the reaction solution was mixed with an equal volume of 10 M urea. The flow-through fraction from the ultrafiltration membrane VIVASPIN 500 MWCO 3000 (Sartorius) was loaded on a SUPELCOSIL LC-18-T (SIGMA-ALDRICH) column and the contents were eluted by 0.1 M potassium phosphate (pH 5.5) at a flow rate of 0.55 ml min −1 . In all, 25 μM cytosine, a saturated concentration of guanine and 50 μM of thymine and adenine in 0.1 M potassium phosphate buffer (pH 5.5) were used as controls. The eluted bases were detected by the absorbance at 260 nm. Mass spectrometry DNA duplex (10 μM) that was used for the co-crystallization and R.PabI dimer (10 μM) were mixed in 100 μl of 10 mM MES (pH 6.0), 300 mM NaCl and 10 mM MgCl 2 and incubated at 40 °C or 85 °C for 1 h. The reaction products were purified by using a QIAquick Nucleotide Removal kit (QIAGEN) before the mass spectrometry analyses. A matrix solution containing 97 mg ml −1 3-hydroxy 2-pyridinecarboxylic acid and 16 mg ml −1 ammonium citrate dibasic in 50% acetonitrile (0.5 μl) was pipetted onto a sample target and mixed with an equal amount of the product DNAs. The samples were analysed with a MALDI-TOF MS AXIMA-CFR Plus (Shimadzu) in the positive reflection mode. Electrophoretic mobility shift assay The 5′-fluorescein-labelled 24-mer DNA duplex described above was used for EMSA assays. Fluorescein-labelled DNA duplex (0.2 μM) and R.PabI dimer (0–1.6 μM) were mixed in the presence of a 25-fold excess amount of an unlabelled competitor DNA duplex (5′-GATGCATGAGATCGAGGACCATC-3′) and incubated in 0.1 M sodium phosphate buffer (pH 6.5) for 30 min at 4 °C. Bound and unbound DNAs were separated through a 12% polyacrylamide gel in 0.5 × TBE at 4 °C and fluorescence was measured by an LAS4000 Mini system. More than 90% of the labelled DNA remained uncleaved after the addition of R.PabI under the conditions used in the EMSA assay. Heat-promoted β elimination of the R.PabI product A total of 4 μM of the 5′-fluorescein-labelled 24-mer DNA duplex described above and 12 μM of the R.PabI dimer were mixed in 100 μl of 10 mM MES (pH 6.0), 300 mM NaCl and 10 mM MgCl 2 and incubated at 40 °C for 1 h. The reaction products were purified by a QIAquick Nucleotide Removal kit (QIAGEN) to remove R.PabI from the solution. To determine the level of heat-promoted β elimination of the R.PabI product, 0.2 μM of the R.PabI product in 0.1 M sodium phosphate buffer (pH 6.5) was incubated at 85 °C. The samples were collected at selected time points and immediately cooled on ice. The fractions of cleaved DNA were visualized by a denaturing 18% polyacrylamide gel as described above. DNA-cleavage assay A modified pET26b plasmid, which has only one 5′-GTAC-3′ site in the lacI -coding sequence, was used as a substrate for R.PabI. The modified pET26b was cut with HindIII (TAKARA) before use to linearize the plasmid. The cleavage by R.PabI splits this 5,360-bp DNA duplex into two DNA fragments of 1,089 bp and 4,271 bp, respectively. To compare the DNA-cleavage activities of the wild-type R.PabI and the K154A mutant, 0.2 μg of R.PabI and 0.2 μg of the substrate DNA were mixed in 20 μl of 0.1 M sodium phosphate buffer (pH 6.5) and incubated at 85 °C for 30 min. To analyse the cleavage of R.PabI products by E. coli lysate, the E. coli JM109 strain (genotype: end A1, rec A1, gyr A96, thi , hsd R17(rk − , mk + ), rel A1, sup E44, Δ( lac - pro AB), (F′ tra D36, pro AB, laq I q ZΔM15)) was cultivated in LB medium until the optical density of the medium at 600 nm reached 1.1. The cells were then collected by centrifugation and lysed by BugBuster (Novagen). The lysate was stored on ice until use. Twenty-microlitre aliquots of the reaction solutions were prepared by mixing 0.2 μg of R.PabI, 0.2 μg of the substrate DNA and 3 μl of BugBuster solution with or without E. coli extract in 0.1 M sodium phosphate buffer (pH 6.5) and incubated at 37 °C for 1 h. The cleaved DNAs were separated by electrophoresis through a 1% agarose gel and visualized with blue-LED light after GelGreen (Biotium) staining. Products by RsaI, which cleaves the DNA duplex at the same site as R.PabI, were also separated as a control. Accession code: Coordinates and structural factors are deposited in the Protein Data Bank under the accession number 3WAZ . How to cite this article: Miyazono, K. et al. A sequence-specific DNA glycosylase mediates restriction-modification in Pyrococcus abyssi . Nat. Commun. 5:3178 doi: 10.1038/ncomms4178 (2014).